The origin of segmentation motor activity in the intestine The segmentation motor activity of the gut that facilitates absorption of nutrients was first described in the late 19th century, but the fundamental mechanisms underlying it remain poorly understood. The dominant theory suggests alternate excitation and inhibition from the enteric nervous system. Here we demonstrate that typical segmentation can occur after total nerve blockade. The segmentation motor pattern emerges when the amplitude of the dominant pacemaker, the slow wave generated by interstitial cells of Cajal associated with the myenteric plexus (ICC-MP), is modulated by the phase of induced lower frequency rhythmic transient depolarizations, generated by ICC associated with the deep muscular plexus (ICC-DMP), resulting in a waxing and waning of the amplitude of the slow wave and a rhythmic checkered pattern of segmentation motor activity. Phase–amplitude modulation of the slow waves points to an underlying system of coupled nonlinear oscillators originating in the networks of ICC. The small intestine of the gastrointestinal tract exhibits two fundamental motor patterns: peristalsis, causing propulsion to move content in anal direction, and segmentation, causing mixing to promote absorption of nutrients and water. We understand much about mechanisms of propulsion [1] , [2] , [3] , [4] but little about segmentation, although it is the most common motor pattern in the small intestine. Intestinal motility is essential for life: when normal motility fails as with intestinal ileus or chronic intestinal pseudo-obstruction, malabsorption and bacterial overgrowth occurs, thereby leading to disabling digestive symptoms and failure to maintain body weight, and treatment may require parenteral nutrition [5] . As segmentation motor patterns are poorly documented and poorly understood, the role of abnormal segmentation in motility disorders [6] is not known, thus negatively impacting attempts to develop appropriate treatments. Propulsive motor activity or peristalsis is now recognized to result from an interplay between interstitial cells of Cajal (ICC) and the enteric nervous system [1] , [7] , [8] . ICC are the intestinal pacemaker cells [2] , [9] , [10] responsible for rhythmic propagation of circular muscle contractions involved in peristalsis [1] . ICC are mesenchymal cells originating from the same precursors as circular smooth muscle cells [11] and here we regard them as part of the myogenic control system of gut motility. Abnormalities in ICC networks are increasingly recognized as being associated with dysfunction of peristalsis [12] , [13] , [14] , [15] . The present study provides a novel mechanism involving ICC in the control of segmentation. The term segmentation is sometimes used to describe any non-propulsive motor activities of the gut but here we refer to segmentation as a specific and characteristic motor pattern originally described in 1902 by Cannon, using X-rays to visualize the motions of the intestine [16] . This specific segmentation motor pattern has the appearance of a ‘checkered pattern’ and is completely distinct from propulsive activity. The mechanism underlying segmentation motor patterns in the small intestine has been proposed to be the alternating inhibition and excitation of smooth muscle by the enteric nervous system [17] , [18] , [19] . We show here that segmentation can occur in the presence of nerve blockade, and we provide evidence for a different mechanism that involves two networks of ICC. Specifically, we demonstrate that the checkered segmentation motor pattern is orchestrated by modulatory phase–amplitude coupling of two interacting pacemaker activities. The amplitude of the slow-wave activity of ICC associated with the myenteric plexus (ICC-MP) is modulated by the phase of lower frequency rhythmic transient depolarizations originating from ICC associated with the deep muscular plexus (ICC-DMP). We hypothesize that induction of rhythmic transient depolarizations in the ICC-DMP changes a propulsive motor pattern into a segmentation motor pattern. Segmentation occurring after nerve conduction block We define segmentation here as a specific and characteristic motor pattern originally described by Cannon [16] . This segmentation occurs when the intestine divides into many sections owing to simultaneous transient contractions, and when these contractions subside, contractions appear more or less at the sites in between the original contractions giving a checkered appearance. This specific segmentation motor pattern occurs in vivo as shown in Fig. 1a , using spatio–temporal maps of the segmentation activity of the mouse intestine; it is distinctly different from peristalsis ( Fig. 1b ) and has a striking similarity to the drawings of Cannon [16] ; Cannon’s drawing is reproduced here in Fig. 1c and can be compared with Fig. 1d , which is a section of Fig. 1a , but turned 90° so that distance and time are aligned with Cannon’s drawing. 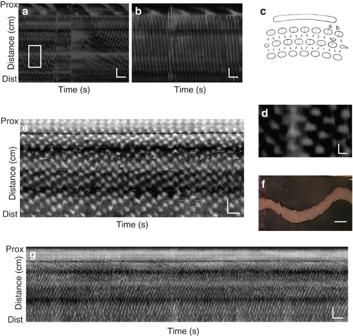Figure 1: Segmentation activity in the intestine in the presence of nerve blockade. (a) Spatio–temporal map ofin vivomouse small intestine segmentation contractions. We describe it here as a checkered pattern, very similar to the original description of Cannon (c). The top shows stomach peristaltic contractions. White represents narrowing of the lumen caused by circular muscle contraction in this and subsequent figures. Scale bars, 0.5 cm, 5 s. Rectangle identifies the section enlarged ind. (b) Spatio–temporal map ofin vivomouse small intestine peristaltic activity. Typical propulsive contractions are seen at the slow-wave frequency of 32 c.p.m. The top shows stomach peristaltic contractions. Scale bars, 0.5 cm, 5 s. (c) The segmentation motor pattern as drawn by Cannon16. Reproduced with permission. From Cannon's original description: A length of mass of food (top line) is cut into a series of uniform segments (2nd line). A moment later each of these segments is divided into two particles (along dotted lines inaandb). Then neighbouring particles merge to form new segments (aandbform intoc). (d) A section cut out of panelaand turned 90 degrees for direct comparison with the drawing from Canon (c). Scale bars, 1 cm, 1 s. (e) Spatio–temporal map of segmentation motor activity in the isolated whole-mouse intestine in the presence of TTX (1 μM). Scale bars, 1 cm, 1 s. (f) Still image from the intestine from whichewas derived. Scale bar, 1 cm. (g) Spatio–temporal map of segmentation motor activity from the same experiment as panele, but displayed for a longer period of time. Scale bars, 1 cm, 10 s. Figure 1: Segmentation activity in the intestine in the presence of nerve blockade. ( a ) Spatio–temporal map of in vivo mouse small intestine segmentation contractions. We describe it here as a checkered pattern, very similar to the original description of Cannon ( c ). The top shows stomach peristaltic contractions. White represents narrowing of the lumen caused by circular muscle contraction in this and subsequent figures. Scale bars, 0.5 cm, 5 s. Rectangle identifies the section enlarged in d . ( b ) Spatio–temporal map of in vivo mouse small intestine peristaltic activity. Typical propulsive contractions are seen at the slow-wave frequency of 32 c.p.m. The top shows stomach peristaltic contractions. Scale bars, 0.5 cm, 5 s. ( c ) The segmentation motor pattern as drawn by Cannon [16] . Reproduced with permission. From Cannon's original description: A length of mass of food (top line) is cut into a series of uniform segments (2nd line). A moment later each of these segments is divided into two particles (along dotted lines in a and b ). Then neighbouring particles merge to form new segments ( a and b form into c ). ( d ) A section cut out of panel a and turned 90 degrees for direct comparison with the drawing from Canon ( c ). Scale bars, 1 cm, 1 s. ( e ) Spatio–temporal map of segmentation motor activity in the isolated whole-mouse intestine in the presence of TTX (1 μM). Scale bars, 1 cm, 1 s. ( f ) Still image from the intestine from which e was derived. Scale bar, 1 cm. ( g ) Spatio–temporal map of segmentation motor activity from the same experiment as panel e , but displayed for a longer period of time. Scale bars, 1 cm, 10 s. Full size image Our first clue to understanding the mechanism of segmentation was the observation of a perfect segmentation motor pattern in the presence of nerve conduction blockade by tetrodotoxin (TTX; 1 μM) ( Fig. 1e–g ; Supplementary movie 1 ). The motor pattern occurred when the whole intestine was submerged in Krebs solution in vitro . The segmental contractions occurred at the slow-wave frequency without neural influence; hence, a myogenic mechanism must underlie segmentation, and the pacemaker system was our first focus of attention. Decanoic acid induced segmentation and waxing and waning In order to investigate segmentation, we found that the nutrient decanoic acid (1 mM) reliably changed a peristaltic motor pattern ( Fig. 2a,b ) into a checkered segmentation motor pattern ( Fig. 2c–e ). To see this, the whole intestine was submerged in an organ bath with intraluminal pressure sensors, extracellular suction electrodes and simultaneous video recording ( n =7). Before the addition of decanoic acid, rhythmic propulsive contractions of similar amplitude at the slow-wave frequency of 34±2 c.p.m. ( Fig. 2a,b ) dominated in all experiments. Extracellular electrical recording obtained at the same time showed that the amplitude of the slow wave was relatively constant ( Fig. 2f ). Decanoic acid evoked the checkered segmentation motor pattern ( Fig. 2c ) associated with segmental divisions of the intestine ( Fig. 2e ). We discovered that the diameter profile (intestinal diameter over time at any one point) of the spatio–temporal maps showed waxing and waning of the amplitude of contraction ( Fig. 2d ); importantly, the electrical slow-wave activity, the signature of pacemaker activity from the ICC-MP, accompanying the segmentation motor activity recorded by extracellular electrodes, also showed a dramatic pattern of waxing and waning ( Fig. 2g ), which was consistent with the observed waxing and waning of the amplitude of the intraluminal pressure transients measured simultaneously ( Fig. 2h ). 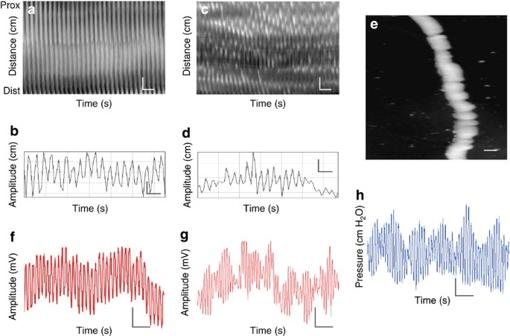Figure 2: Association between segmentation and waxing and waning patterns. (a) Spatio–temporal map shows normal propulsive motor pattern of the rat intestine before addition of decanoic acid. Scale bars, 0.5 cm, 5 s. (b) Amplitude profile (degree of narrowing of the lumen) taken at one point of the intestine showing regular amplitude contractions over time. Scale bars, 0.2 cm, 4 s. (c) Spatio–temporal map of segmentation motor activity evoked by addition of 1 mM decanoic acid. Scale bars, 0.5 cm, 5 s. (d) Amplitude profile frombshowing waxing and waning. Scale bars, 0.2 cm, 4 s. (e) Still image related tocshowing multiple contractions of the intestine dividing it into segments in the presence of decanoic acid. Scale bar, 1 cm. (f) Extracellular electrical recording obtained at the same time as activity shown ina. The amplitude of the slow wave is relatively constant. Scale bars, 1 mV, 20 s. (g) Extracellular electrical activity obtained at the same time as activity shown incshows a waxing and waning pattern during segmentation activity. Scale bars, 1 mV, 20 s. (h) Simultaneously measured intraluminal pressure shows waxing and waning in amplitude during segmental activity shown inc. Scale bars, 0.5 cm H2O, 20 s. Figure 2: Association between segmentation and waxing and waning patterns. ( a ) Spatio–temporal map shows normal propulsive motor pattern of the rat intestine before addition of decanoic acid. Scale bars, 0.5 cm, 5 s. ( b ) Amplitude profile (degree of narrowing of the lumen) taken at one point of the intestine showing regular amplitude contractions over time. Scale bars, 0.2 cm, 4 s. ( c ) Spatio–temporal map of segmentation motor activity evoked by addition of 1 mM decanoic acid. Scale bars, 0.5 cm, 5 s. ( d ) Amplitude profile from b showing waxing and waning. Scale bars, 0.2 cm, 4 s. ( e ) Still image related to c showing multiple contractions of the intestine dividing it into segments in the presence of decanoic acid. Scale bar, 1 cm. ( f ) Extracellular electrical recording obtained at the same time as activity shown in a . The amplitude of the slow wave is relatively constant. Scale bars, 1 mV, 20 s. ( g ) Extracellular electrical activity obtained at the same time as activity shown in c shows a waxing and waning pattern during segmentation activity. Scale bars, 1 mV, 20 s. ( h ) Simultaneously measured intraluminal pressure shows waxing and waning in amplitude during segmental activity shown in c . Scale bars, 0.5 cm H 2 O, 20 s. Full size image Intracellular recording of waxing and waning To avoid any potential motion artefacts in the electrical recordings, we also recorded intracellular electrical activity to assess the absolute membrane potential changes in mechanically fixed pieces of intestine. We observed at the submucosal side of the circular muscle layer that decanoic acid changed regular, constant amplitude slow-wave activity into a waxing and waning pattern ( Fig. 3a ) ( n =10). The waxing and waning electrical activity was noted previously by Diamant and Bortoff [20] and Suzuki et al. [21] who suggested that it might be caused by interaction of two slow waves from the same pacemaker network (ICC-MP) occurring at slightly different frequencies. Indeed, when we superimposed (summated) two sine waves resembling slow-wave activities of slightly different frequency, a waxing and waning pattern emerged; however, the amplitude of the largest oscillation was twice that of the original slow-wave amplitude; and in our experiments with decanoic acid, there was no significant change in amplitude. Furthermore, it has been shown using arrays of a few 100 electrodes that when two slow waves within the same network interact, one of them will be annihilated when hitting the refractory period of the other slow wave [22] . Hence, interaction of two slow waves from within the same pacemaker network is unlikely to generate an ongoing segmentation motor pattern. 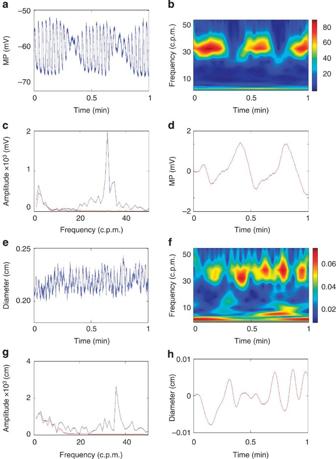Figure 3: Continuous wavelet transform (CWT) analysis of slow-wave activity and segmentation. (a) Intracellular electrical activity of circular muscle in the presence decanoic acid (1 mM). MP, membrane potential. (b) Time–frequency contour plot of mean power (CWT analysis) shows a high-frequency component (~32 cycles per min) with a low-frequency component (~3 cycles per min) in source signala. Red and blue indicate a power increase or decrease, respectively. (c) Fourier transform (FFT) analysis of signal a shows complete frequency distribution of source signal (blue) and filtered low-frequency signal (red). (d) Signal filtering shows the presence of a low oscillatory activity in the source signal (a). Note that high-frequency power inbis time-locked to the trough of the filtered low-frequency signal ind. MP, membrane potential. (e) Diameter changes over time obtained from the spatio–temporal map (amplitude profile) in the presence of decanoic acid at one point along the intestine. (f) Time–frequency contour plot of mean power of source signal (e) (CWT analysis) shows the high-frequency (~38 cpm) signal amplitude with significant low-frequency signals throughout (~5 c.p.m). Red and blue indicate a power increase or decrease, respectively. (g) FFT analysis of signal (e) shows complete frequency distribution of source signals (blue) and filtered low-frequency signals (red). (h) Significant low-frequency signal shows after filtering source signal (e). Note that high-frequency power infis time-locked to the trough of the filtered low-frequency signal inh. The low frequency is not stationary. Figure 3: Continuous wavelet transform (CWT) analysis of slow-wave activity and segmentation. ( a ) Intracellular electrical activity of circular muscle in the presence decanoic acid (1 mM). MP, membrane potential. ( b ) Time–frequency contour plot of mean power (CWT analysis) shows a high-frequency component (~32 cycles per min) with a low-frequency component (~3 cycles per min) in source signal a . Red and blue indicate a power increase or decrease, respectively. ( c ) Fourier transform (FFT) analysis of signal a shows complete frequency distribution of source signal (blue) and filtered low-frequency signal (red). ( d ) Signal filtering shows the presence of a low oscillatory activity in the source signal ( a ). Note that high-frequency power in b is time-locked to the trough of the filtered low-frequency signal in d . MP, membrane potential. ( e ) Diameter changes over time obtained from the spatio–temporal map (amplitude profile) in the presence of decanoic acid at one point along the intestine. ( f ) Time–frequency contour plot of mean power of source signal ( e ) (CWT analysis) shows the high-frequency (~38 cpm) signal amplitude with significant low-frequency signals throughout (~5 c.p.m). Red and blue indicate a power increase or decrease, respectively. ( g ) FFT analysis of signal ( e ) shows complete frequency distribution of source signals (blue) and filtered low-frequency signals (red). ( h ) Significant low-frequency signal shows after filtering source signal ( e ). Note that high-frequency power in f is time-locked to the trough of the filtered low-frequency signal in h . The low frequency is not stationary. Full size image Continuous wavelet transform analysis We wished to further understand the frequency characteristics of the segmentation activity, and so we performed both continuous wavelet transform (CWT) and Fourier transform (FFT) analysis on the electrical and the motor activity recordings. CWT allows analysis of non-stationary frequency activity over time. CWT analysis of the intracellularly recorded waxing and waning pattern of the circular muscle electrical activity in the presence of decanoic acid showed both a high-frequency activity at ~32 cycles per min ( Fig. 3b,c ) as well as a strong oscillatory activity at about 3 cycles per min ( Fig. 3b,d ). Consistently, recordings of the intestinal diameter over time (that is, the profiles of segmentation motor patterns, Fig. 3e ) showed similar frequency characteristics, namely 38 and 5 cycles per min ( Fig. 3f–h ). FFT analysis was concordant with the CWT analysis ( Fig. 3f,g ). Origin of the low-frequency component To identify the source of the frequency components, we used live calcium imaging of the mouse intestinal tissue. Tissues were focussed at different depths, ICC-MP were identified by their multipolar shape, whereas ICC-DMP are elongated cells running parallel to circular muscle cells. C-kit staining (red) showed ICC-MP ( Fig. 4a ), a layer in between ICC-MP and ICC-DMP ( Fig. 4b ) and ICC-DMP ( Fig. 4c ) using fluorescence microscopy. The ICC-MP ( Fig. 4a ) showed rhythmic calcium transients ( Fig. 4d,e ) as shown previously [23] at the same frequency as the omnipresent slow-wave activity recorded in electrical recordings consistent with previous studies [24] . We were not certain about the origin of the low-frequency component. We therefore investigated the possibility that the second network of ICC in the small intestine, the ICC that are distributed between the inner and outer parts of the circular muscle layer at the level of the deep muscular plexus, the ICC-DMP, might be the source. Calcium oscillatory activity in ICC-DMP showed quiescence ( n =12) or low-frequency calcium oscillations (2–5 c.p.m., n =6). The low-frequency calcium oscillations were particularly prominent in the presence of decanoic acid (1 mM) ( Fig. 4f,g ). Thus, we hypothesized that the low-frequency electrical activity identified by CWT analysis in the musculature originated from ICC-DMP, and we termed this activity as rhythmic transient depolarizations. 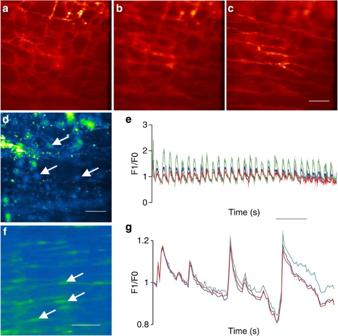Figure 4: ICC in the small intestine harbour high- and low-frequency activities. Live tissue c-kit staining (red) of ICC-MP (a), the layer in between ICC-MP and ICC-DMP (b) and ICC-DMP (c) using fluorescence microscopy. This is the same tissue focussed at different depths. ICC-MP are identified by their multipolar shape, whereas ICC-DMP are elongated cells running parallel to circular muscle cells. (d) The Fluo-4 calcium signal was recorded in the presence of decanoic acid (1 mM). ICC-MP show spontaneous calcium oscillations at 30 c.p.m. (e) From the three cells indicated by arrows ind, the intensity (F1/F0) versus time is shown. (f) ICC-DMP show calcium oscillations at 4 c.p.m. in the presence of decanoic acid (1 mM). (g) From the three cells indicated by arrows inf, the intensity (F1/F0) versus time is shown. Scale bars,a–d,f, 20 μm;e,g, 10 s Figure 4: ICC in the small intestine harbour high- and low-frequency activities. Live tissue c-kit staining (red) of ICC-MP ( a ), the layer in between ICC-MP and ICC-DMP ( b ) and ICC-DMP ( c ) using fluorescence microscopy. This is the same tissue focussed at different depths. ICC-MP are identified by their multipolar shape, whereas ICC-DMP are elongated cells running parallel to circular muscle cells. ( d ) The Fluo-4 calcium signal was recorded in the presence of decanoic acid (1 mM). ICC-MP show spontaneous calcium oscillations at 30 c.p.m. ( e ) From the three cells indicated by arrows in d , the intensity (F1/F0) versus time is shown. ( f ) ICC-DMP show calcium oscillations at 4 c.p.m. in the presence of decanoic acid (1 mM). ( g ) From the three cells indicated by arrows in f , the intensity (F1/F0) versus time is shown. Scale bars, a – d , f , 20 μm; e , g , 10 s Full size image Modulatory phase–amplitude coupling The slow-wave activity of the ICC-MP and the rhythmic transient depolarizations of the ICC-DMP will propagate into the musculature. The next question we wished to pursue concerned how the low- and high-frequency oscillations interacted to create the waxing and waning pattern in electrical activity measured in the musculature and to create the motor pattern of segmentation. To investigate the nature of the interaction between the low- and high frequencies, we looked to the brain literature, wherein cross-frequency coupling is a well-studied phenomenon [25] , [26] , [27] . Cross-frequency coupling involves the interaction of one timescale or frequency component of a signal with a different timescale or frequency component. Such coupling is often described as some interaction between amplitudes or phases. The amplitude of the rhythmic signal associated with one frequency may be modulated by the phase of the rhythmic signal associated with another frequency (phase–amplitude coupling) [25] , the amplitude of one frequency may be modulated by a change in amplitude of another frequency (amplitude–amplitude coupling) or the phases of the two frequencies may have a consistent relationship (phase–phase coupling) [28] . The appearance of waxing and waning of the slow-wave activity in intracellular electrical recordings of smooth muscle was not accompanied by a change in amplitude of the high-frequency activity, making modulation of the amplitude of the higher frequency by the amplitude of the lower unlikely. We likewise did not see clear evidence for phase–phase coupling, as the phases of the two rhythms did not seem consistently aligned over time. We therefore hypothesized that the high-frequency activity’s amplitude may instead be modulated by the phase of the lower frequency. This is commonly referred to as phase–amplitude coupling [25] , [26] , [27] . We used a technique known as the modulation index (MI; see Methods) to investigate such phase–amplitude coupling. Strong phase–amplitude coupling was observed in the electrical coupling of the low and high-frequency activities observed in the intracellular electrical activity of the circular muscle layer ( Fig. 5a–f ), as shown by the high and significant value of the MI. Importantly, recordings of the intestine diameter over time (representing rhythmic circular muscle contractions) showed similar phase–amplitude-coupling patterns ( Fig. 5g–l ). Again, the MI showed strong and significant modulation of the amplitude of the high-frequency component by the phase of the low-frequency component. Such modulation can also be appreciated in the time domain as a strengthening of the higher frequency rhythm at specific portions of the phase of the lower frequency rhythm. To demonstrate this, the original time-domain plot of diameter over time was first band-pass filtered from 0.5 to 5 cycles per min to obtain the low-frequency component ( Fig. 5m ). The higher frequency component was obtained by band-pass filtering from 30 to 50 cycles per min and was superimposed on the lower frequency signal ( Fig. 5n ). There was a clear relationship between the phase of the lower frequency signal and the amplitude of the higher frequency signal. 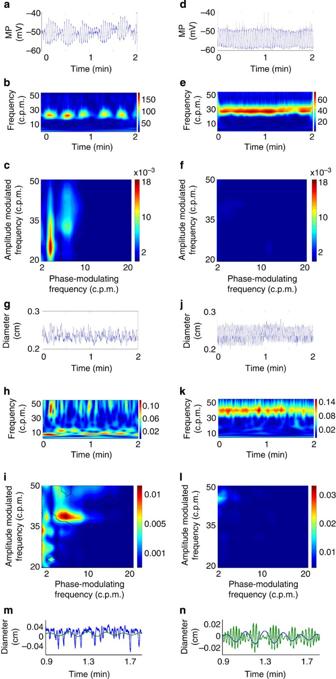Figure 5: Assessment of modulatory amplitude–phase coupling. (a) Waxing and waning of electrical slow-wave activity in the presence of decanoic acid (1 mM); 2 min recording. MP, membrane potential. (b) Time–frequency contour plot of mean power (continuous wavelet transform analysis) ofashows high (~25 c.p.m.) and low-(~3 c.p.m.) frequency components. (c) Modulation index (MI) of the phase–amplitude coupling (see Methods). Modulation of the higher frequency (~25 c.p.m.) component’s amplitude by the phase of a lower frequency (~3 c.p.m.) component is measured, where higher values (towards red) indicate greater modulation. Areas within black lines indicate significance with an alpha value of 0.05 using surrogate methods. (d) Intracellular electrical activity of circular muscle in the absence of decanoic acid. MP, membrane potential. (e) Time–frequency contour plot of mean power shows the high-frequency (~30 cycles per min) signal without significant low-frequency signals throughout. (f) No modulation (see Methods) is apparent, as no low-frequency component is present ind. (g) Waxing and waning pattern of intestine diameter recorded at one point along the small intestine during segmentation activity (2 min recording). (h) Time–frequency contour plot of mean power ofg. (i) MI carried out as inc. Highly significant modulation of the higher frequency (38 c.p.m.) component’s amplitude by the phase of a lower frequency (~4 c.p.m.) is seen. (j) Constant amplitude intestine diameter recorded at one point along the small intestine during propulsion activity (2 min recording). (k) Time–frequency contour plot of mean power shows the high frequency (~38 c.p.m.) signal amplitude without significant low-frequency signals throughout. (l) No significant modulation is seen because of lack of significant low-frequency components. (m) To further demonstrate the nature of the cross-frequency coupling in the segmentation waxing and waning pattern ofg, part ofgdepicted here (0.9–1.7 min) was band-pass filtered between 0.5 and 5 cycles per min to obtain the low-frequency component as shown. (n) The higher frequency component from the signal inmwas obtained by band-pass filtering from 30 to 50 cycles per min and was superimposed on the lower frequency signal. A clear relationship is seen between the phase of the lower frequency and the amplitude of the higher frequency. Figure 5: Assessment of modulatory amplitude–phase coupling. ( a ) Waxing and waning of electrical slow-wave activity in the presence of decanoic acid (1 mM); 2 min recording. MP, membrane potential. ( b ) Time–frequency contour plot of mean power (continuous wavelet transform analysis) of a shows high (~25 c.p.m.) and low-(~3 c.p.m.) frequency components. ( c ) Modulation index (MI) of the phase–amplitude coupling (see Methods). Modulation of the higher frequency (~25 c.p.m.) component’s amplitude by the phase of a lower frequency (~3 c.p.m.) component is measured, where higher values (towards red) indicate greater modulation. Areas within black lines indicate significance with an alpha value of 0.05 using surrogate methods. ( d ) Intracellular electrical activity of circular muscle in the absence of decanoic acid. MP, membrane potential. ( e ) Time–frequency contour plot of mean power shows the high-frequency (~30 cycles per min) signal without significant low-frequency signals throughout. ( f ) No modulation (see Methods) is apparent, as no low-frequency component is present in d . ( g ) Waxing and waning pattern of intestine diameter recorded at one point along the small intestine during segmentation activity (2 min recording). ( h ) Time–frequency contour plot of mean power of g . ( i ) MI carried out as in c . Highly significant modulation of the higher frequency (38 c.p.m.) component’s amplitude by the phase of a lower frequency (~4 c.p.m.) is seen. ( j ) Constant amplitude intestine diameter recorded at one point along the small intestine during propulsion activity (2 min recording). ( k ) Time–frequency contour plot of mean power shows the high frequency (~38 c.p.m.) signal amplitude without significant low-frequency signals throughout. ( l ) No significant modulation is seen because of lack of significant low-frequency components. ( m ) To further demonstrate the nature of the cross-frequency coupling in the segmentation waxing and waning pattern of g , part of g depicted here (0.9–1.7 min) was band-pass filtered between 0.5 and 5 cycles per min to obtain the low-frequency component as shown. ( n ) The higher frequency component from the signal in m was obtained by band-pass filtering from 30 to 50 cycles per min and was superimposed on the lower frequency signal. A clear relationship is seen between the phase of the lower frequency and the amplitude of the higher frequency. Full size image Regeneration of the segmentation motor pattern To provide further evidence that waxing and waning of the segmentation motor pattern is indeed due to phase–amplitude coupling, we obtained experimentally generated low- and high-frequency signals, and reconstituted signals very similar to the original signals seen using a generalizable model of phase–amplitude-coupling activity (see Methods). We started by filtering out the low-frequency component of the activated intracellular electrical activity under decanoic acid ( Fig. 6a,b ) and the high-frequency component of the control electrical activity before decanoic acid administration ( Fig. 6c ). Coupling these two recordings ( Fig. 6b,c ) together (see Methods) generated the waxing and waning pattern ( Fig. 6d ) very similar to the original waxing and waning signal ( Fig. 6a ). We performed similar analysis on the segmentation motor pattern ( Fig. 6e ). The low-frequency components of every position in space of waxing and waning segmentation motor activity under decanoic acid ( Fig. 6f ) were first obtained. High-frequency activity was obtained from all points in space from control propulsive motor patterns ( Fig. 6g ). Phase–amplitude coupling of these two signals provided not only waxing and waning patterns similar to the originals, but also the original segmentation motor activity over space ( Fig. 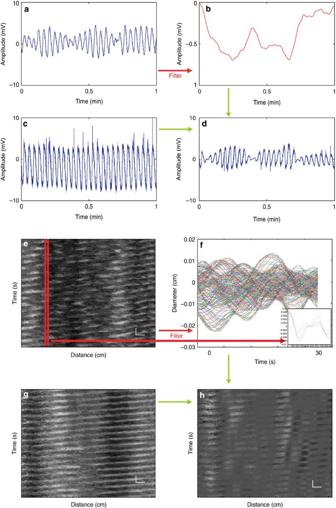Figure 6: Reconstitution of the waxing and waning patterns. Reconstitution of the waxing and waning patterns of electivity activity and the checkered segmentation pattern of motor activity. (a) Intracellular electrical activity in the presence of decanoic acid showing the typical waxing and waning pattern. (b) Low-frequency component ofaobtained by band-pass filtering processing. (c) Typical intracellular electrical activity recorded before the addition of decanoic acid. (d) When the phase of the low-frequency component (b) was coupled to the amplitude of the high-frequency component (c) using modulated phase–amplitude coupling the typical waxing and waning pattern emerged similar to the recording ina. (e) An example of a 3.8-cm section of the intestine exhibiting a segmentation motor pattern for 30 s in the presence of lidocaine (0.5 mM). Scale bars, 0.25 cm, 2 s. (f) At each measured point along the intestine, the amplitude profile (degree of lightness) was taken and filtered to obtain the low-frequency component. The inset shows the low-frequency components of five consecutive positions along the intestine in between the red lines. (g) Propulsive motor patterns before addition of lidocaine, the white bands representing the contractile state are uninterrupted. Scale bars, 0.25 cm, 2 s. (h) Here the reconstituted image is shown where each point in space is constructed using the amplitude profiles of the propulsive motor pattern (g) as the high-frequency amplitude signal source and the corresponding filtered low-frequency component (f) as the low-frequency phase signal source to execute phase–amplitude coupling. The result is a checkered motor pattern that is similar to the recording ine. Scale bars, 0.25 cm, 2 s. 6h ) Figure 6: Reconstitution of the waxing and waning patterns. Reconstitution of the waxing and waning patterns of electivity activity and the checkered segmentation pattern of motor activity. ( a ) Intracellular electrical activity in the presence of decanoic acid showing the typical waxing and waning pattern. ( b ) Low-frequency component of a obtained by band-pass filtering processing. ( c ) Typical intracellular electrical activity recorded before the addition of decanoic acid. ( d ) When the phase of the low-frequency component ( b ) was coupled to the amplitude of the high-frequency component ( c ) using modulated phase–amplitude coupling the typical waxing and waning pattern emerged similar to the recording in a . ( e ) An example of a 3.8-cm section of the intestine exhibiting a segmentation motor pattern for 30 s in the presence of lidocaine (0.5 mM). Scale bars, 0.25 cm, 2 s. ( f ) At each measured point along the intestine, the amplitude profile (degree of lightness) was taken and filtered to obtain the low-frequency component. The inset shows the low-frequency components of five consecutive positions along the intestine in between the red lines. ( g ) Propulsive motor patterns before addition of lidocaine, the white bands representing the contractile state are uninterrupted. Scale bars, 0.25 cm, 2 s. ( h ) Here the reconstituted image is shown where each point in space is constructed using the amplitude profiles of the propulsive motor pattern ( g ) as the high-frequency amplitude signal source and the corresponding filtered low-frequency component ( f ) as the low-frequency phase signal source to execute phase–amplitude coupling. The result is a checkered motor pattern that is similar to the recording in e . Scale bars, 0.25 cm, 2 s. Full size image Absorption of nutrients is the most important function of the intestine, and the segmentation motor pattern is essential for this. Although the enteric nervous system has a critical role in the expression of most intestinal motor activities, we show here that a perfect segmentation motor pattern is easily expressed after total blockade of the enteric nervous system, which implies that a myogenic control system is underlying it. The myogenic control system involves the smooth muscle cells and the ICC. The ICC-MP network generates pacemaker activity, omnipresent slow waves that are transmitted to the circular muscle layer [2] , [9] , [29] . The slow waves are initiated in the proximal intestine and control peristaltic contractions [1] . The role of ICC-DMP is poorly understood, but here we present evidence that this ICC network does not produce omnipresent activity but can produce low-frequency rhythmic transient depolarizations associated with rhythmic changes in intracellular calcium. When these rhythmic transient depolarizations are transmitted into the circular muscle layer, phase–amplitude interaction with the slow-wave activity occurs. This causes a waxing and waning pattern of electrical slow-wave activity ( Fig. 7 ), and consequently a checkered pattern of non-propagating motor activity appears ( Fig. 1 ; Supplementary movie 1 ). Hence, we propose that induced rhythmic transient depolarizations in the ICC-DMP are a critical factor in changing the motor pattern from propulsion to segmentation. Currently, we are investigating which physiological stimuli can evoke segmentation through induction of the rhythmic transient depolarizations in the ICC-DMP. Whether or not a motor pattern occurs in response to nutrients or distention in vivo is often determined by the response of the enteric nervous system to the stimulus. This is most likely also the case for segmentation, and several components of the enteric nervous system have been shown to be involved [30] . This neural activity then works in concert with the ICC pacemaker activities to generate the motor pattern of segmentation. 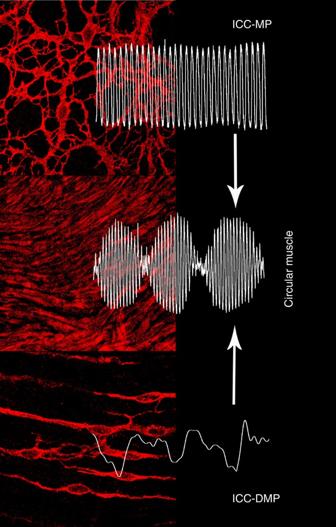Figure 7: Phase–amplitude coupling leads to a waxing and waning slow-wave pattern. Schematic using immunofluorescent images and electrical recordings to show the origin of the electrical pacemaker activities and their interaction in the circular smooth muscle layer. Figure 7: Phase–amplitude coupling leads to a waxing and waning slow-wave pattern. Schematic using immunofluorescent images and electrical recordings to show the origin of the electrical pacemaker activities and their interaction in the circular smooth muscle layer. Full size image We have not yet investigated through what mechanism decanoic acid alters the ICC-DMP activity, but we can speculate that it is through activation of phospholipase C and consequently IP 3 (Inositol trisphosphate)-induced increase in intracellular calcium that would trigger calcium-dependent ion channels to initiate a transient depolarization. This is based on studies in an epithelial cell line in which decanoic acid has been shown to affect paracellular permeability by activating phospholipase C, resulting in an increase in intracellular calcium [31] , [32] . Slow-wave initiation in the ICC-MP is thought to be associated with IP 3 -induced calcium release triggering ion channel activity [23] , [33] , [34] , [35] . Hence, a similar mechanism of IP 3 -mediated induction of transient depolarizations may exist in ICC-DMP. The literature surrounding cross-frequency coupling in the brain is extensive, and is often associated with theories of non-linear-coupled oscillators [25] , [36] , [37] , [38] . Electrical activity in the intestine, in particular the slow-wave activity in the ICC-MP network, has also been discussed in terms of non-linear oscillators [39] , [40] , [41] . As a result of the present study, future work on in silico modelling of the small bowel needs to include at least two non-linear oscillators to better understand the dynamic nature of the intestinal pacemaker system. In summary, both intracellular electrical activity of the circular smooth muscle and segmentation motor activity demonstrate phase–amplitude coupling of a low-frequency component (2–5 cycles per min) with a high-frequency component (30–40 cycles per min). This, combined with the recording of low-frequency activity in the calcium transients of ICC-DMP, and high-frequency activity in the calcium transients of ICC-MP provide evidence for a coordinating role of the two ICC networks in the segmentation motor activity of the mammalian small bowel. This discovery allows us to put a central focus on the role of the ICC in pathology in our ongoing efforts to understand mammalian small bowel motility and dysmotility. Although the ICC have been shown to have a role in motility disorders, their exact role in specific motor abnormalities is still missing. The present study provides direction for efforts to identify morphological and functional roles of the ICC networks in patients with small bowel motility dysfunction. Motility video recording and spatio–temporal mapping CD-1 mice (female, 14 weeks old (Charles River Laboratories International, Inc., Wilmington, MA, USA) were killed by overdose of chloroform followed by exsanguination. All animal procedures were approved by the McMaster University Animal Research Ethics Board. Lengths of small intestine were placed in organ baths containing oxygenated Krebs solution at 36 °C and were imaged with web cameras (Macally, Toronto, Ontario, Canada) mounted above the organ bath at a resolution of 0.014 cm per pixel and 33 ms per frame. Specific conditions (pressurization and drugs added to bath) varied with experiment and are indicated in figure legends. Motility maps were created from web camera recordings with a custom plugin for ImageJ (National Institutes of Health, Bethesda, MD, USA) written by S.P.P. With the length of the intestine parallel to the x axis of the camera frame, the plugin calculates the width of the intestine at each pixel along the x axis by intensity thresholding. This gives an image of intestine width (image intensity) as a function of time ( x axis) and length along the intestine ( y axis). This image is called a ‘motility map’ or ‘spatio–temporal map’. Lighter colours in the map indicate contraction and darker colours indicate relaxation. In order to assess activities in the absence of functional activity of the enteric nervous system, TTX (1 μM) was applied. In the presence of TTX, electrical field stimulation of enteric nerves does not evoke excitatory or inhibitory neural responses [42] . Electrical activity recording of the circular muscle Intracellular recordings were performed on sections of the jejunum from the excised small intestine of adult (14 weeks of age) female CD-1 mice (Charles River Laboratories International, Inc.) immediately after cervical dislocation. Segments were opened along the length of the mesenteric border and pinned flat on a Sylgard gel dish, mucosa facing upwards. Tissue was continuously submerged in oxygenated (95% O 2 , 5% CO 2 ) Krebs solution (118.1 mM NaCl, 1.0 mM NaH 2 PO 4 , 1.2 mM MgSO 4 , 2.5 mM CaCl 2 , 4.8 mM KCl, 11.1 mM glucose, 25 mM NaHCO 3 ) and maintained at room temperature. All recordings were made in the presence of nicardipine (0.5 μM). After the tissue was pinned down, the mucosal and submucosal layers were carefully removed using fine dissection forceps to expose the circular smooth muscle layers. Recordings were obtained from tissue preparations continuously perfused (4 ml min −1 ) with oxygenated Krebs solution at 37 °C viewed under a high-powered inverted microscope (Zeiss Axiovert S100 TV). Intracellular electrical recordings of circular smooth muscle cells were performed by impalement with borosilicate glass micropipettes (fire polished; length: 7 cm; outer diameter: 1.5 mm, inner diameter: 0.86 mm) filled with 3 M KCl and fabricated to yield resistance between 30 and 70 MΩ. We used a MultiClamp 700B amplifier (Axon Instruments) to record electrical signals from smooth muscle. These signals were digitized at an acquisition rate of 2 kHz using an Axon Instruments Digidata 1322A acquisition system Fig. 2a ). Direct current was used with zero intensity (no current was injected) to record membrane potentials of smooth muscle cells near the level of the DMP. Decanoic acid was dissolved in dimethyl sulfoxide to create a stock solution of 1 M. This ensured that as little DMSO as possible was added to the Krebs solution (1/1,000 dilution). This dilution of DMSO did not have an effect on the electrical activities. Stable recordings of slow waves (at least 5 min) were challenged with addition of 1 mM decanoic acid. To obtain control activity again after decanoic acid treatment, decanoic acid was flushed out with fresh oxygenated Krebs solution. Lidocaine was dissolved in dimethyl sulfoxide or ethanol dimethyl sulfoxide, and the solvent did not create the demonstrated effects. Nicardipine (0.5 μM) was dissolved in fresh Krebs. Extracellular electrical activity was measured using a platinum electrode touching the outside of the rat intestine amplified through EGG equipment (MedKinetic, Ningbo, China). Whole-rat intestines were placed in organ baths in the same way as reported for studies on the rat colon [7] . These studies were approved by the ethics committee of Renmin Hospital of Wuhan University. Calcium imaging of the ICC-MP and ICC-DMP Tissue preparation for calcium imaging of ICC-DMP activity was the same as for the intracellular microelectrode recording of the circular musculature of the mouse intestine (see above described). Fine forceps were used to peel off strips of circular muscle bundles until a few ganglia with surrounding ICC-MP were clearly exposed. Tissue was equilibrated in oxygenated Krebs solution for ~0.5–1 h before use. Fluo-4-AM calcium imaging was used to visualize calcium oscillations in the ICC-MP and ICC-DMP. A 2.5-mM stock solution of Fluo-4-AM dye (Molecular Probes, Burlington, Ontario, Canada) was prepared in DMSO and 20% Pluronic F-127 and used within a week. The tissue preparation was incubated with a final concentration of 5 μM fluo-4-AM and 0.02% Pluronic F-127 in 1.5 ml oxygenated Krebs solution for 20 min, and then perfused with oxygenated Krebs solution for 20–30 min before imaging to allow for full de-esterification of AM esters. To determine whether the cells exhibiting calcium oscillation were in fact ICC, c-Kit staining was carried out. ACK2 (rat anti-mouse c-kit antibody; (14–1172) eBiosciences, San Diego, CA, USA) was conjugated to Alexa Fluor 594 (Alexa Fluor 594 Monoclonal Antibody Labeling Kit (A-20185); Molecular Probes) before staining. Tissue preparation was incubated with 5 g ml −1 ACK2-Alexa Fluor 594 in 1 ml Krebs solution for 1 h at 4 °C. Fluo-4 loading as described above was performed after 20–30 min. Imaging was carried out on a Nikon Eclipse FN-S2N upright fluorescence microscope. Water immersion × 40 objectives with a GFP filter and a Lambda DG-4 illuminator (Sutter Instrument Co., Novato, CA, USA) were used to excite Alexa Fluor 594 and Fluo-4, dyes with peak excitation wavelengths of 594 and 488 nm, respectively. Images were captured using a Quantum 512SC camera with a frame rate of 5–10 frames per second and Nikon-NIS Elements imaging software. Recordings of calcium transients over time were analysed using the Nikon-NIS elements program. Borders of ICC were traced to create region of interests (ROIs). Three or more ICC were analysed for each experiment. The fluorescence intensity was presented as the ratio F1/F0 in which the raw fluorescence intensity signals of a ROI were compared with the first fluorescence signal in that ROI. ROIs were selected by eye and traced by hand and encompassed the cell body of the ICC to be analysed. The frequency was presented as the number of signal peaks per minute, analysed using Clampfit or Excel. CWT and FTT frequency analysis All analysis was implemented in MATLAB (version 7.12.0 (R2011a). The raw signals from one recording of intracellular electrical activity (1 min, 250 ms sampling interval) and from one position over time of spatio–temporal mapping (1 min, 33 ms sampling interval) were used for further spectral analysis. Two standard signal processing techniques, namely the CWT and the FFT, were used to transform the signals from the time domain into the frequency domain, allowing the analysis of the spectral content of our signals. For the CWT, we chose to use the morlet wavelet transform [43] with a centre frequency of 0.8125 and a frequency bandwidth of 5. The CWT is a particularly useful technique as it allows analysis of frequency over time, thereby providing an ability to understand the nature of non-stationary, dynamic aspects of a signal of interest. Modulation index Many processes in biology consist of rhythmical activity coupled across multiple frequency scales. One common regime in which such coupling exists is referred to as phase–amplitude modulation wherein the phase of a lower frequency signal dictates the amplitude of a higher frequency signal. Often the amplitude of the higher frequency signal is concentrated on only one portion of the phase of the lower frequency signal. Description of such activity is ubiquitous in the brain literature and several signal processing techniques have been devised (see, for example, Tort et al. [26] and Canolty et al. [27] ). We chose to use the technique of Tort et al. [26] as it has greater reliability overall. This technique uses a measure from information theory called the Kulback–Liebler entropy (KLE). The KLE is a metric for the ‘distance’ between two probability distributions P (·) and Q (·) (ref. 44 ). Let x be a random variable with a set of possible states { x }, then the KLE is defined as: In particular, MI involves the binning of amplitude estimates ( AMP ) of the higher frequency component of a signal over the phase ( ϕ ) of a lower frequency component of a signal. A pseudo-probability distribution ( AMP { ϕ bin }) is obtained by normalizing the binned amplitudes and is compared by the KLE to a uniform distribution ( U { ϕ bin }) over the same phases. The MI is then obtained by normalization by log (N) , assuring that the metric varies from 0 to 1 (ref. 26 ): In order to run more rigorous statistics, we chose to further test the values of MI by surrogate methods. We used the amplitude-adjusted FFT (AAFT) surrogate technique introduced by Theiler et al. [45] . This method scrambles the phase of the lower frequency signal while keeping its autocorrelogram or, equivalently, its spectral density, constant. 200 AAFT surrogate phase signals are created and the MI calculation is computed 200 times using the surrogate data. A P value is then obtained by comparison of the original value of MI with that obtained over the distribution of MI values obtained using the surrogate data [45] . Signal reconstructions using amplitude–phase coupling To supplement the amplitude–phase-coupling analysis, signal reconstruction from component signals was achieved. The Hilbert transform can be used to generate a complex analytic signal x analytic from a real signal x : Where is the Hilbert transform of x . The Hilbert transform was used in order to extract the phase estimates ( φ(x) ) from the lower frequency portion of the signal (band-pass filtered from 2 to 8 c.p.m.) and the amplitude estimates from the higher frequency portion of the signal using standard definitions of phase and amplitude in the complex plane. As the analytic signal can equivalently be expressed as: The signal can be reconstructed using amplitude and phase estimates alone. If we assume that the signal is well described by the phase estimate of a lower frequency and the amplitude estimate of a higher frequency, then the corresponding signal reconstruction would be: where the higher and lower frequency signals are referred to as X L and X H , respectively. Note that this form makes use of the same assumptions used in the MI. How to cite this article: Huizinga, J. D. et al. The origin of segmentation motor activity in the intestine. Nat. Commun. 5:3326 doi: 10.1038/ncomms4326 (2014).